Observation of topologically protected bound states in photonic quantum walks Topological phases exhibit some of the most striking phenomena in modern physics. Much of the rich behaviour of quantum Hall systems, topological insulators, and topological superconductors can be traced to the existence of robust bound states at interfaces between different topological phases. This robustness has applications in metrology and holds promise for future uses in quantum computing. Engineered quantum systems—notably in photonics, where wavefunctions can be observed directly—provide versatile platforms for creating and probing a variety of topological phases. Here we use photonic quantum walks to observe bound states between systems with different bulk topological properties and demonstrate their robustness to perturbations—a signature of topological protection. Although such bound states are usually discussed for static (time-independent) systems, here we demonstrate their existence in an explicitly time-dependent situation. Moreover, we discover a new phenomenon: a topologically protected pair of bound states unique to periodically driven systems. Phases of matter have long been characterized by their symmetry properties, with each phase classified according to the symmetries that it possesses [1] . The discovery of the integer and fractional quantum Hall effects in the 1980s has led to a new paradigm, where quantum phases of matter are characterized by the topology of their ground-state wavefunctions. Since then, topological phases have been identified in physical systems ranging from condensed-matter [2] , [3] , [4] , [5] , [6] , [7] , [8] , [9] and high-energy physics [10] to quantum optics [11] and atomic physics [12] , [13] , [14] , [15] . Topological phases of matter are parametrized by integer topological invariants. As integers cannot change continuously, a consequence is exotic phenomena at the interface between systems with different values of topological invariants. For example, a topological insulator supports conducting states at the surface, precisely because its bulk topology is different to that of its surroundings [8] , [9] . Creating and studying new topological phases remains a difficult task in a solid-state setting because the properties of electronic systems are often hard to control. Using controllable simulators may be advantageous in this respect. Here we simulate one-dimensional topological phases using a discrete time quantum walk [16] , a protocol for controlling the motion of quantum particles on a lattice. We create regions with distinct values of topological invariants and directly image the wavefunction of bound states at the boundary between them. The controllability of our system allows us to make small changes to the Hamiltonian and demonstrate the robustness of these bound states. Finally, using the quantum walk, we can access the dynamics of strongly driven systems far from the static or adiabatic regimes [17] , [18] , [19] , to which most previous work on topological phases has been restricted. In this regime, we discover a topologically protected pair of non-degenerate bound states, a phenomenon that is unique to periodically driven systems. Split-step quantum walks Discrete time quantum walks have been realized in several physical architectures [20] , [21] , [22] , [23] , [24] . Here we use the photonic set-up demonstrated in ref. 24 to implement a variation of these walks, the split-step quantum walk [25] of a single photon, with two internal states encoded in its horizontal, | H 〉, and vertical, | V 〉, polarization states. The quantum walk takes place on a one dimensional lattice ( Fig. 1 ). One step of the split-step quantum walk consists of four steps. First, a polarization rotation R ( θ 1 ) of the single photon is achieved with a suitable wave plate (see Methods ), then a polarization-dependent translation T 1 of | H 〉 to the right by one lattice site using a calcite beam displacer. This is followed by a second rotation R ( θ 2 ), and finally another translation T 2 of | V 〉 to the left. The quantum walk is implemented by repeated applications of the one-step operator U ( θ 1 , θ 2 )= T 2 R ( θ 2 ) T 1 R ( θ 1 ). 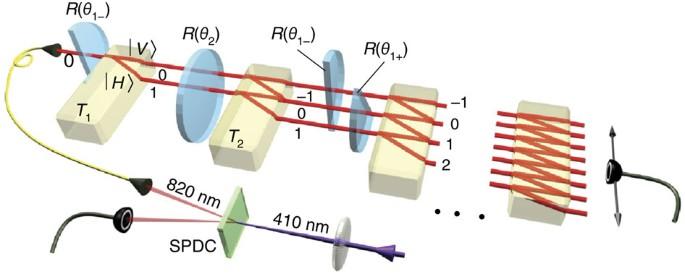Figure 1: Experimental scheme for split-step quantum walks. A polarization-encoded single photon, created via spontaneous parametric downconversion (SPDC), undergoes a succession of steps consisting of polarization rotations,R(θ1),R(θ2), and translations,T1,T2, which displace |H〉 and |V〉, respectively. The rotations are implemented by half-wave plates while the translations are implemented using birefringent calcite beam displacers. To probe the topological properties of the quantum walk, semi-circular half-wave plates are used to create spatially inhomogeneous rotations,R(θ1−),R(θ1+). The output probability distribution is imaged with a single-photon avalanche detector. Figure 1: Experimental scheme for split-step quantum walks. A polarization-encoded single photon, created via spontaneous parametric downconversion (SPDC), undergoes a succession of steps consisting of polarization rotations, R ( θ 1 ), R ( θ 2 ), and translations, T 1 , T 2 , which displace | H 〉 and | V 〉, respectively. The rotations are implemented by half-wave plates while the translations are implemented using birefringent calcite beam displacers. To probe the topological properties of the quantum walk, semi-circular half-wave plates are used to create spatially inhomogeneous rotations, R ( θ 1− ), R ( θ 1+ ). The output probability distribution is imaged with a single-photon avalanche detector. Full size image The propagation of the photon in the static experimental set-up can be described by an effective time-dependent Schrödinger equation with periodic driving. The dynamics of the quantum walk can be understood through the effective Hamiltonian H eff ( θ 1 , θ 2 ), defined through where τ is the time required for one step of the quantum walk. Throughout this paper, we chose units such that Therefore, the quantum walk described by the evolution U ( θ 1 , θ 2 ) corresponds to a stroboscopic simulation of the effective Hamiltonian H eff ( θ 1 , θ 2 ) viewed at unit time intervals. That is, after n steps of the quantum walk, the photon evolves according to meaning that the evolution under the quantum walk coincides with the evolution under H eff ( θ 1 , θ 2 ) for integer multiples of τ . The topological structure underlying split-step quantum walks is revealed by studying the structure and symmetry of H eff ( θ 1 , θ 2 ). H eff ( θ 1 , θ 2 ) has a gapped spectrum, with two bands corresponding to opposite polarizations ( Fig. 2a ). Because the quantum walk is translationally invariant, each eigenstate is associated with a quasi-momentum k and a superposition of | H 〉 and | V 〉. In addition, this class of quantum walks has a chiral symmetry described in ref. 25 (also detailed in the Methods), which requires that the polarization component of any eigenstate be confined to a particular great circle on the Bloch sphere. Therefore, as the quasi-momentum k traverses the first Brillouin zone from − π to π , the polarization component of the eigenstate traces a closed path confined to that great circle, see Fig. 2b and Methods. The total number of times W that this closed path winds about the origin is the winding number and gives the topological invariant of H eff ( θ 1 , θ 2 ). 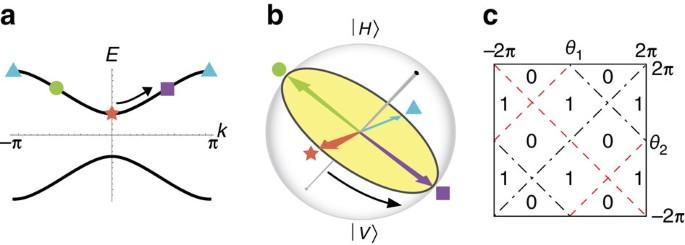Figure 2: Band structure and phase diagram of split-step quantum walks. (a) A typical band structure of the effective HamiltonianHeff(θ1,θ2) for the split-step quantum walk (here,θ1=π/2 andθ2=0). For mostθ1andθ2, the spectrum displays a gap. (b) Topology ofHeff(θ1,θ2). Each eigenstate ofHeff(θ1,θ2) consists of a quasi-momentumkand a corresponding polarization, shown here on a Bloch sphere using the symbols froma. Askruns from −πtoπ(black arrow ina), the polarization follows a closed trajectory around a great circle (black arrow inb). The winding number of this trajectory,W, characterizes the topology ofHeff(θ1,θ2). (c) Phase diagram ofHeff(θ1,θ2) that shows the winding numberWas a function ofθ1andθ2. The transition lines correspond to points where the spectral gap ofHeff(θ1,θ2) closes at eigenvaluesE=0 (black dash-dotted line) andE=π(red dashed line). Figure 2: Band structure and phase diagram of split-step quantum walks. ( a ) A typical band structure of the effective Hamiltonian H eff ( θ 1 , θ 2 ) for the split-step quantum walk (here, θ 1 = π /2 and θ 2 =0). For most θ 1 and θ 2 , the spectrum displays a gap. ( b ) Topology of H eff ( θ 1 , θ 2 ). Each eigenstate of H eff ( θ 1 , θ 2 ) consists of a quasi-momentum k and a corresponding polarization, shown here on a Bloch sphere using the symbols from a . As k runs from − π to π (black arrow in a ), the polarization follows a closed trajectory around a great circle (black arrow in b ). The winding number of this trajectory, W , characterizes the topology of H eff ( θ 1 , θ 2 ). ( c ) Phase diagram of H eff ( θ 1 , θ 2 ) that shows the winding number W as a function of θ 1 and θ 2 . The transition lines correspond to points where the spectral gap of H eff ( θ 1 , θ 2 ) closes at eigenvalues E =0 (black dash-dotted line) and E = π (red dashed line). Full size image Because W has to be an integer, it cannot be changed by small modifications of the effective Hamiltonian. That is, W can only change when the spectrum of H eff ( θ 1 , θ 2 ) closes its gap while preserving chiral symmetry. For the split-step quantum walk, two distinct topological phases with W =0 and W =1 exist as can be seen in the phase diagram shown in Fig. 2c . The two phases are separated by lines along which the gap closes. As we mentioned above, non-trivial topological phases support localized states at their boundaries. Because our experimental set-up allows access to individual lattice sites, we can probe this phenomenon by creating a boundary between regions where the dynamics are governed by two different gapped Hamiltonians H eff ( θ 1− , θ 2 ) and H eff ( θ 1+ , θ 2 ), characterized by winding numbers W − and W + respectively. We create the boundary by making θ 1 spatially inhomogeneous with θ 1 ( x )= θ 1− for lattice positions x <0 and θ 1 ( x )= θ 1+ for x ≥0. Although this breaks translational symmetry, the chiral symmetry remains (see Methods ). When W − ≠ W + , it is expected that topologically robust localized states exist at the boundary near x =0. This can be understood in a heuristic fashion as follows. When W − ≠ W + , the winding number W − of the bulk gapped Hamiltonian H eff ( θ 1− , θ 2 ) can only be changed to that of H eff ( θ 1+ , θ 2 ) given by W + by closing the gap of the system. Thus, near the boundary between these two regions, the energy gap closes, and it is expected that states exist within the gaps of the bulk spectra of H eff ( θ 1− , θ 2 ) and H eff ( θ 1+ , θ 2 ). Because extended states do not exist inside the gap, such a state is necessarily localized at the boundary. That is, a change in topology at a boundary is accompanied by the presence of a localized state. Furthermore, we are able to show that the localized states are robust against perturbations [26] such as small changes of quantum walk parameters or the presence of a static disordered potential caused by, for example, small spatial variations of rotation angles θ 1 and θ 2 . Experimental confirmation of bound states To probe the existence of the bound states, we initialize a photon next to the boundary between two topologically distinct quantum walks ( Fig. 1 ). In the absence of bound states, the photon is expected to spread ballistically, with the detection probability at the origin quickly decreasing to zero. However, if there is a bound state, the bound state component of the initial state will remain near this boundary even after many steps. We first implemented split-step quantum walks with θ 2 = π /2 and θ 1− and θ 1+ such that W − = W + =1, as shown on the phase diagram in Fig. 3a . For initial photon polarizations of | H 〉 and | V 〉, shown in Fig. 3b,c respectively, the detection probability at the origin quickly decreases to zero. On the other hand, in Fig. 3d , with parameters chosen to create a boundary between topologically distinct phases W − =0 and W + =1, we observe the existence of at least one bound state as a peak in the probability distribution near the origin after four steps. 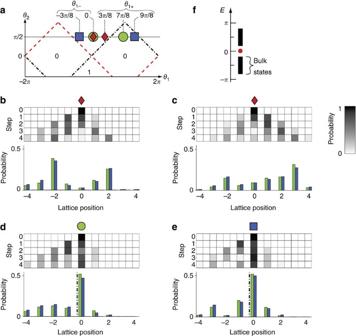Figure 3: Experimental quantum walks with topologically protected bound states. (a) Phase diagram, with symbols indicating the parameters (θ1−,θ1+,θ2), and the corresponding winding numbers for each experimental case (b–e). (b–e) Experimental probability distributions of split-step quantum walks forθ2=π/2 and a spatially inhomogeneous rotationR(θ1). The probabilities of finding the photon at a particular site are indicated by the shading in the upper panel. The bar graphs below each dataset compare the measured (blue) and predicted (green) probabilities after the fourth step. Experimental errors due to photon counting statistics are not visible on this scale. (b) and (c) show the absence of a bound state nearx=0 for initial polarizations |H〉 and |V〉 respectively. (d) Initial polarization of |H〉, the presence of a bound state with a pronounced peak nearx=0 after the fourth step. The phase boundary is indicated on the bar plot by the dash-dotted black line. (e) Initial polarization of |H〉, the presence of the bound state is robust against changes to the parameters ind. (f) Calculated quasi-energy spectrum of the effective Hamiltonian ford. The bound state with quasi-energyE=0 is indicated by the red dot. Figure 3: Experimental quantum walks with topologically protected bound states. ( a ) Phase diagram, with symbols indicating the parameters ( θ 1− , θ 1+ , θ 2 ), and the corresponding winding numbers for each experimental case ( b – e ). ( b – e ) Experimental probability distributions of split-step quantum walks for θ 2 = π /2 and a spatially inhomogeneous rotation R ( θ 1 ). The probabilities of finding the photon at a particular site are indicated by the shading in the upper panel. The bar graphs below each dataset compare the measured (blue) and predicted (green) probabilities after the fourth step. Experimental errors due to photon counting statistics are not visible on this scale. ( b ) and ( c ) show the absence of a bound state near x =0 for initial polarizations | H 〉 and | V 〉 respectively. ( d ) Initial polarization of | H 〉, the presence of a bound state with a pronounced peak near x =0 after the fourth step. The phase boundary is indicated on the bar plot by the dash-dotted black line. ( e ) Initial polarization of | H 〉, the presence of the bound state is robust against changes to the parameters in d . ( f ) Calculated quasi-energy spectrum of the effective Hamiltonian for d . The bound state with quasi-energy E =0 is indicated by the red dot. Full size image We note that our experiment is able to detect bound states with fewer steps than the theoretical study in ref. 25 , because we use a sharper boundary between distinct topological phases. As a result, the bound states become narrower and are more easily detected. We can test the robustness of these bound states against a variety of changes in microscopic parameters to confirm that they are topologically protected. In Fig. 3e , θ 1− and θ 1+ are shifted from those of Fig. 3d while maintaining W − =0 and W + =1, and we confirmed the continued existence of a bound state. The quasi-energy E of this localized state, that is, the eigenvalue of the effective Hamiltonian associated with this state, can be found by explicit calculation ( Fig. 3f ). We indeed find a single state at E =0. Observation of pairs of bound states in quantum walks Our experiment also reveals a new topological phenomenon unique to periodically driven systems, which can be probed by studying split-step quantum walks with θ 2 =0, and the θ 1 parameters shown in Fig. 4a . With the appropriate choice of basis (see Methods ), this quantum walk becomes equivalent to the one described by the one-step operator U=iTR ( θ 1 ), where T = T 1 T 2 can be implemented with a single calcite beam displacer, extending the experiment to seven steps. This class of quantum walks can only realize a single topological phase characterized by the winding number W =0. Therefore, we do not expect bound states for spatially inhomogeneous θ 1 based on winding numbers. However, the evolution of the probability distribution shown in Fig. 4b displays period-2 oscillations in the vicinity of the origin. This observation strongly suggests the existence of at least two bound states whose quasi-energies differ by π . 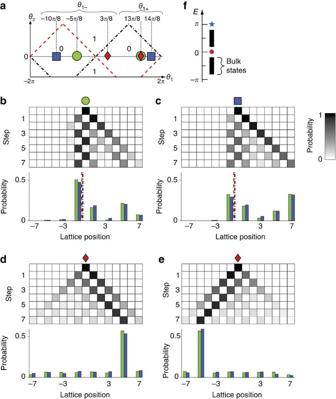Figure 4: Experimental quantum walks with a pair of topologically protected bound states. (a) Phase diagram, with symbols indicating the parameters (θ1−,θ1+,θ2), and corresponding winding numbers for each experimental case (b–e). (b–e) Experimental probability distributions of split-step quantum walks forθ2=0 and a spatially inhomogeneous rotationR(θ1). The probabilities of finding the photon at a particular site are indicated by the shading in the upper panel. The bar graphs below each dataset compare the measured (blue) and predicted (green) probabilities after the seventh step. Experimental errors due to photon counting statistics are not visible on this scale. (b) Initial polarization |H〉. A pair of bound states with period-2 oscillations are present and there is a large probability of detecting the photon near the boundary after seven steps. The phase boundary is indicated on the bar plot by both the dash-dotted black and dashed red lines. (c) Initial polarization |H〉. Small perturbations made to the quantum walk parameters ofbdo not change the topology and therefore the bound states remain. (d) and (e) show the absence of a bound state nearx=0 for initial polarizations |H〉 and |V〉, respectively. (f) Quasi-energy spectrum of the effective Hamiltonian forb. In addition to theE=0 (red dot) bound state there is anE=πbound state (blue star). Figure 4: Experimental quantum walks with a pair of topologically protected bound states. ( a ) Phase diagram, with symbols indicating the parameters ( θ 1− , θ 1+ , θ 2 ), and corresponding winding numbers for each experimental case ( b – e ). ( b – e ) Experimental probability distributions of split-step quantum walks for θ 2 =0 and a spatially inhomogeneous rotation R ( θ 1 ). The probabilities of finding the photon at a particular site are indicated by the shading in the upper panel. The bar graphs below each dataset compare the measured (blue) and predicted (green) probabilities after the seventh step. Experimental errors due to photon counting statistics are not visible on this scale. ( b ) Initial polarization | H 〉. A pair of bound states with period-2 oscillations are present and there is a large probability of detecting the photon near the boundary after seven steps. The phase boundary is indicated on the bar plot by both the dash-dotted black and dashed red lines. ( c ) Initial polarization | H 〉. Small perturbations made to the quantum walk parameters of b do not change the topology and therefore the bound states remain. ( d ) and ( e ) show the absence of a bound state near x =0 for initial polarizations | H 〉 and | V 〉, respectively. ( f ) Quasi-energy spectrum of the effective Hamiltonian for b . In addition to the E =0 (red dot) bound state there is an E = π bound state (blue star). Full size image Again, we can demonstrate that these bound states are robust against small perturbations to the walk parameters. The parameters for Fig. 4c are chosen so that they are continuously connected with those for Fig. 4b . As expected, we observe the period-2 oscillations in the evolution of probability distributions indicating the existence of a pair of bound states whose quasi-energies differ by π . We confirm the absence of bound states for split-step quantum walks with θ 2 =0 when θ 1− and θ 1+ are continuously connected without crossing a phase boundary. The results in Fig. 4d,e show detection probabilities that quickly decrease to zero near the boundary for initial polarizations | H 〉 and | V 〉, respectively. As | H 〉 and | V 〉 span the space of internal states for the walker, this shows that indeed there is no bound state near x =0. The existence of a pair of bound states with quasi-energy difference π is a previously unknown topological phenomenon. It is a consequence of chiral symmetry, defined as the existence of an operator Γ that anti-commutes with the Hamiltonian, Γ H Γ −1 =− H . An eigenstate | ψ 〉 with energy E therefore implies the existence of an eigenstate Γ −1 | ψ 〉 with energy − E . That is, states with energies E and − E generally come in pairs—the only exception is if E = −E . In a static system, a single state with energy zero can exist because its energy satisfies E =− E (ref. 26 ). It is topologically protected: it cannot be shifted in energy by weak, symmetry-preserving perturbations because a single state cannot be split into two. In a periodically driven system, because the effective Hamiltonian is defined through a one-step evolution operator by the quasi-energies of H eff ( θ 1 , θ 2 ) are defined only up to 2 π . In particular, E = π and E =− π correspond to the same quasi-energy, and, therefore, E = π represents another special value of quasi-energy satisfying E =− E . Thus, like zero-energy states of static systems, a single state with quasi-energy π is topologically protected [17] , [18] . The coexistence of E =0 and E = π states suggested by the period-2 oscillations, observed in Fig. 4b , is verified through the explicit calculation of the quasi-energy spectrum presented in Fig. 4f . In the Methods section, we give the characterisation of this structure in terms of topological invariants of periodically driven systems and prove their topological robustness. Bound states under decoherence One feature of our optical quantum walk set-up is the ability to tune the level of decoherence [24] . Each pair of beam displacers forms an interferometer, which can be intentionally misaligned to add temporal and spatial walk-off [24] . This process, coupled with measurement of the photon, corresponds well to pure dephasing [24] . If the system at step N is described by the density matrix ρ N , it will evolve according to: where p is the amount of dephasing and K i are the associated Kraus operators. For p =0, equation 1 describes a pure quantum walk, while p =1 represents a system without any quantum coherence, that is, the evolution is described by a classical random walk. Although p =0 indicates that we do not introduce deliberate dephasing, some may arise from experimental imperfections. Although the topological bound states observed in the paper are no longer eigenstates of the quantum walk under dephasing, signatures of bound states are still observable for a small number of steps. This result demonstrates that it is possible to study topological phenomena, for short times, in other systems that might be more prone to decoherence. In Fig. 5 , we show split-step quantum walks with θ 1 and θ 2 parameters equivalent to those presented in Fig. 4b,d . However, here we have introduced additional decoherence at a level of p =0.2 according to equation 1. Fig. 5a shows the same period-2 oscillation as before demonstrating that a pair of bound states can be seen with this small amount of decoherence. The absence of a bound state is confirmed when we chose W − = W + =0, and the results are shown in Fig. 5b . 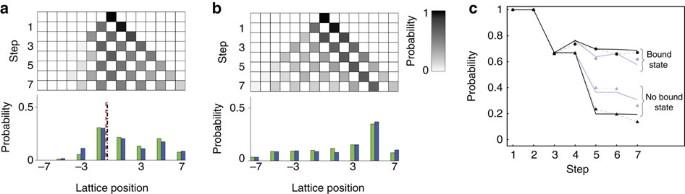Figure 5: Paired bound states in the presence of decoherence. (a,b) Probability distributions for split-step quantum walks with additional decoherence,p=0.2, for the initial polarization state |H〉. The probabilities of finding the photon at a particular site are indicated by the shading in the upper panel and the bar graphs below each dataset compare the measured (blue) and predicted (green) probabilities after the seventh step. Experimental errors due to photon counting statistics are not visible on this scale. For these walksθ2=0 andR(θ1) is spatially inhomogeneous. (a) A pair of bound states is observed between two distinct topological phases despite the added decoherence. The phase boundary is indicated on the bar plot by both the dash-dotted black and dashed red lines. (b) Absence of bound states in the presence of decoherence. (c) Sum of probabilities at lattice positions around the boundary (−1, 0 and +1) for integer steps of the split-step quantum walks with and without bound states. The solid lines show theoretical predictions and the dashed lines are the experimental results, error bars are smaller than the marker size. The difference between bound and unbound states can be seen for both datasets, with no added decoherence (black), and with added decoherence (blue). Figure 5: Paired bound states in the presence of decoherence. ( a , b ) Probability distributions for split-step quantum walks with additional decoherence, p =0.2, for the initial polarization state | H 〉. The probabilities of finding the photon at a particular site are indicated by the shading in the upper panel and the bar graphs below each dataset compare the measured (blue) and predicted (green) probabilities after the seventh step. Experimental errors due to photon counting statistics are not visible on this scale. For these walks θ 2 =0 and R ( θ 1 ) is spatially inhomogeneous. ( a ) A pair of bound states is observed between two distinct topological phases despite the added decoherence. The phase boundary is indicated on the bar plot by both the dash-dotted black and dashed red lines. ( b ) Absence of bound states in the presence of decoherence. ( c ) Sum of probabilities at lattice positions around the boundary (−1, 0 and +1) for integer steps of the split-step quantum walks with and without bound states. The solid lines show theoretical predictions and the dashed lines are the experimental results, error bars are smaller than the marker size. The difference between bound and unbound states can be seen for both datasets, with no added decoherence (black), and with added decoherence (blue). Full size image In the presence of dephasing, the bound state observed in Fig. 4b gradually decays as the number of steps increases. However, for slow dephasing, this decay is slow and, for few steps, the probability distribution is still peaked near the boundary compared with the cases with no bound states ( Fig. 5a ). Fig. 5c summarizes the effect of decoherence on the probability distribution around the boundary region). The bound states observed in Fig. 3d,e are direct analogues of the zero-energy states in the Su-Schrieffer-Heeger (SSH) model of polyacetylene [27] and the Jackiw-Rebbi model of a one-dimensional spinless Fermi field coupled to a Bose field [10] . Specifically, the SSH model describes conduction in conjugated organic polymers, of which polyacetylene is the simplest example. By studying this polymer from a topological perspective, they identified the formation of a 'topological soliton' [27] that is responsible for the charge-transfer doping mechanism in this molecule. Despite these theoretical predictions, its topological nature has never directly been confirmed. With our system, we have simulated the same class of topological phases as the SSH model and demonstrated their robustness to system perturbations for the first time. The experiment can be extended to other symmetry classes and higher dimensions. In particular, the beam displacer architecture could also implement a two-dimensional walk [28] , which would allow observation of topologically protected edge states. Furthermore, one could simulate many topological classes of static systems that have been theoretically predicted but have not yet been realized because of the lack of natural materials with suitable symmetries [25] . In addition, novel topological phenomena, unique to periodically driven systems, are expected in other symmetry classes and dimensions. The versatility of photonic quantum walks makes them ideal tools for exploring these captivating phenomena [17] . Rotation operators implemented in the experiment The implementation of split-step quantum walks with a photon requires the rotations of polarization, written as R ( θ ). In this experiment, we used half-wave plates that implement where σ i are the Pauli matrices such that σ z | H 〉=| H 〉 and σ z | V 〉=−| V 〉. Winding numbers of split-step quantum walk In our theoretical proposal [25] , we considered creating a boundary between regions with different topological numbers by varying the second rotation angle θ 2 . We described the topological structure of the split-step quantum walk in terms of the one-step evolution operator, or Floquet operator, U ( θ 1 , θ 2 )= T 2 R ( θ 2 ) T 1 R ( θ 1 ) and associated chiral symmetry operator which depends only on θ 1 and satisfies In this experiment, we implemented inhomogeneous split-step quantum walks by varying the first rotation angle, θ 1 . To maintain the chiral symmetry in the system, it is necessary to characterize the dynamics in terms of an alternative chiral symmetry operator that depends only on the second rotation angle, θ 2 . In the following, we explain and define such a chiral symmetry operator. As a consequence of considering such a chiral symmetry operator, the present phase diagrams are slightly different from those in ref. 25 . Because the origin of time for a periodically driven system is arbitrary, we can characterize the topology of the split-step quantum walk with a different initial time, namely in terms of the evolution operator U′ ( θ 2 , θ 1 )= T 1 R ( θ 1 ) T 2 R ( θ 2 ). This alternative choice corresponds to making a half-period shift of the origin of time. Using the momentum-space expressions and we see that U′ ( θ 2 , θ 1 ) is different from U ( θ 1 , θ 2 ) only through the exchange of θ 1 and θ 2 , that is, U′ ( θ 2 , θ 1 )= U ( θ 1 , θ 2 ). Therefore, it is clear that the chiral symmetry operator of U′ ( θ 2 , θ 1 ) is given by and that the winding numbers of U′ ( θ 2 , θ 1 ) are the same as those of U ( θ 1 , θ 2 ). The chiral symmetry of U′ ( θ 2 , θ 1 ) only depends on the second rotation angle θ 2 , and thus the symmetry is preserved even when θ 1 is varied in space. Therefore, it is possible to construct inhomogeneous quantum walks with boundaries between topologically distinct phases, while preserving the required chiral symmetry across the entire system. The split-step quantum walk with θ 2 =0 We studied the behaviour of the split-step quantum walk U = T 2 R ( θ 2 ) T 1 R ( θ 1 ) with θ 2 =0, noting that R ( θ =0)= σ z . In the experiment, we implemented the quantum walk with Floquet operator U ex = T 2 T 1 R ( θ 1 ). In this section, we show that these two quantum walks are related through a unitary transformation, and therefore represent equivalent dynamics with equivalent topological properties. The split-step quantum walk with θ 2 =0 is described by the Floquet operator It is simple to check that the unitary transformation acts on T=T 2 T 1 such that V −1 TV = iTσ z , where ^ is the coordinate operator. Therefore, U ( θ 1 , 0) and U ex are unitarily related through Apart from a global phase, the experimental implementation is equivalent to the split-step quantum walk with θ 2 =0. Topological invariants of 0 and π energy bound states In this section, we show that the topological classification of periodically driven systems with chiral symmetry is given by Z×Z , and give explicit expressions for the topological invariants in terms of the wavefunctions of the bound states. These invariants provide another way to understand the topological protection of the 0- and π -energy bound states found in the experiment. We consider the bound states at energy 0 because analogous arguments apply to the bound states at π . Suppose that there are N 0 degenerate bound states with energy 0, which we label with α ′=1,..., N 0 . Because the chiral symmetry operator Γ anticommutes with the Hamiltonian, Γ 2 commutes with H . When there is no conserved quantity [29] associated with Γ 2 , it is possible to choose the phase of Γ such that Γ 2 =1. Because is an eigenstate of H with energy 0, we can choose the basis of zero-energy states such that they are eigenstates of Γ . We denote the zero-energy states in this basis as | ψ α 0 〉 and their eigenvalues under Γ as Q α 0 . As Γ 2 =1, Q α 0 is either +1 or −1. We now show that the sum of eigenvalues, the integer represents the topological invariant associated with zero-energy bound states. The invariant Q π for π -energy bound states is constructed in an analogous fashion, where | ψ α π 〉 are the π -energy bound states. To show that these quantities are indeed topological invariants, we show that perturbations to the Hamiltonian that preserve the chiral symmetry cannot mix the zero- and π -energy bound states with the same eigenvalues of Γ , and therefore cannot change the energies of these states away from 0 or π . Let H ′ be a perturbation to the system such that { Γ , H ′}=0. Now we evaluate the matrix element of { Γ , H ′}=0 between the 0 ( π ) energy states. The result is Thus, bound states with the same eigenvalues Q α cannot mix, whereas those with different eigenvalues in general do mix and are not protected by chiral symmetry. Because one can break up any finite change of the Hamiltonian into successive changes of small perturbations, one can repeat this argument and show that the values Q 0 and Q π cannot change unless the bound states at 0 and π energies mix with the bulk states. In the limiting case of the split-step quantum with θ 2 =0, θ 1− =−π, θ 1 = π , we can analyse the bound states of the shifted evolution operator U′ ( θ 2 , θ 1 )= T 1 R ( θ 1 ) T 2 with chiral operator The bound-state wavefunctions can be easily computed and one finds a single zero-energy bound state with Q 0 =1 and a single π -energy bound state with Q π =−1. Because the pair of bound states found in the experiment arises in a situation that is continuously connected with this limiting split-step quantum walk without closing the gaps, the observed pair is characterized by the same values of the topological invariants. How to cite this article: Kitagawa, T. et al . Observation of topologically protected bound states in photonic quantum walks. Nat. Commun. 3:882 doi: 10.1038/ncomms1872 (2012).